Unique domain appended to vertebrate tRNA synthetase is essential for vascular development New domains were progressively added to cytoplasmic aminoacyl transfer RNA (tRNA) synthetases during evolution. One example is the UNE-S domain, appended to seryl-tRNA synthetase (SerRS) in species that developed closed circulatory systems. Here we show using solution and crystal structure analyses and in vitro and in vivo functional studies that UNE-S harbours a robust nuclear localization signal (NLS) directing SerRS to the nucleus where it attenuates vascular endothelial growth factor A expression. We also show that SerRS mutants previously linked to vasculature abnormalities either deleted the NLS or have the NLS sequestered in an alternative conformation. A structure-based second-site mutation, designed to release the sequestered NLS, restored normal vasculature. Thus, the essential function of SerRS in vascular development depends on UNE-S. These results are the first to show an essential role for a tRNA synthetase-associated appended domain at the organism level, and suggest that acquisition of UNE-S has a role in the establishment of the closed circulatory systems of vertebrates. Aminoacyl transfer RNA (tRNA) synthetases (aaRSs) are enzymes essential for translation throughout the three kingdoms of life [1] , [2] . Each member of the tRNA synthetase family is responsible for charging one specific amino acid onto its cognate tRNA. Once the tRNA is charged and delivered to the ribosome, the amino acid can be transferred from the tRNA onto a growing peptide according to the genetic code. During the evolution of this ancient protein family, new domains and motifs were progressively added to aaRSs to expand their functionalities [3] , [4] , [5] , [6] . These appended domains, often dispensable for aminoacylation, are considered as markers for the aaRS-associated functions beyond translation [6] . Although their appearance correlates with the increase of biological complexity in higher organisms, the functional significance of these aaRS-associated appended domains is not understood at the organism level. With this question in mind, we recently identified a unique domain (named UNE-S) at the carboxyl-terminus of seryl-tRNA synthetase (SerRS) in all vertebrates from fish to humans [6] . Interestingly, three independent forward-genetic studies in zebrafish suggested a role for SerRS in vascular development [7] , [8] , [9] . Disruption of the gene encoding the cytoplasmic SerRS by insertional mutagenesis results in a null mutation, and causes abnormal blood vessel formation and defective blood circulation in the embryo [7] . Separately, two additional studies identified three N -ethyl- N -nitrosourea-induced mutations in SerRS that also cause vasculature defects [8] , [9] . Two of these mutations result in premature stop codons (Q402Stop and E421Stop) eliminating part of the aminoacylation domain and the entire UNE-S domain, while the third is a missense mutation (F383V) located in the aminoacylation domain and allows expression of the full enzyme. Microinjection of either human or zebrafish SerRS messenger RNA (mRNA) into ko095 (Q402Stop) mutant zebrafish embryos rescued the vascular phenotype, indicating that the vascular role of SerRS is conserved between zebrafish and humans [8] . Interestingly, an aminoacylation-defective SerRS (T429A SerRS) mRNA could also restore the vasculature phenotype, suggesting that the role of SerRS in vasculature development is independent of aminoacylation [8] . This noncanonical activity of SerRS was linked to the expression of vegfa , the gene encoding vascular endothelial growth factor A (VEGFA), a key regulator of angiogenesis and vasculogenesis [8] . Considering that UNE-S was joined to SerRS at the time of development of the closed circulatory system, we speculated that UNE-S is relevant to the noncanonical role of SerRS in vascular development. In this study, we identified a nuclear localization signal (NLS) sequence embedded in UNE-S, and designed a series of experiments to demonstrate that the essential role of SerRS in vascular development is dependent on UNE-S and its role to mobilize SerRS from the cytoplasm to the nucleus. UNE-S-dependent nuclear localization of SerRS From inspection of UNE-S, we identified a KKQKK QXEXX KKK sequence as a putative NLS sequence that is highly conserved in all vertebrates ( Fig. 1 ). This observation raised the possibility that, in addition to being present in the cytoplasm for protein synthesis, SerRS might also be distributed to the nucleus. Confocal immunofluorescence microscopy demonstrated nuclear localization of SerRS in human endothelial cells (that is, HUVECs) ( Fig. 2a ). Cell fractionation analysis further confirmed the nuclear distribution of SerRS in HUVECs ( Fig. 2b ). Nuclear distribution of endogenous SerRS was also detected in HEK 293 T cells ( Fig. 2b ), indicating that the mechanism for bringing SerRS into the nucleus is not restricted to endothelial cells. We estimated that for both cell types, ∼ 10% of cellular SerRS is located in the nucleus based on our western blot analysis ( Fig. 2b ). 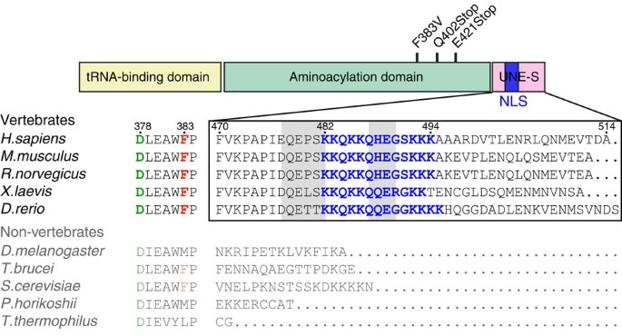Figure 1: Domain structure of vertebrate SerRS and the appearance of the UNE-S domain during evolution. Mutations causing vasculature abnormalities in zebrafish are labelled on top of the domain structure. The sequence segments D378-F383 and F470-A514 of human SerRS are aligned with the same regions from other vertebrates and non-vertebrates SerRS sequences. The predicted nuclear localization signal sequence (NLS) embedded in the UNE-S domain is highlighted in blue. Figure 1: Domain structure of vertebrate SerRS and the appearance of the UNE-S domain during evolution. Mutations causing vasculature abnormalities in zebrafish are labelled on top of the domain structure. The sequence segments D378-F383 and F470-A514 of human SerRS are aligned with the same regions from other vertebrates and non-vertebrates SerRS sequences. The predicted nuclear localization signal sequence (NLS) embedded in the UNE-S domain is highlighted in blue. 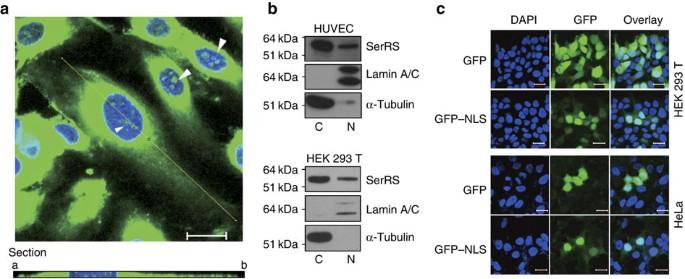Figure 2: Nuclear localization of SerRS. (a) Confocal immunofluorescence microscopy showing the nuclear localization of the endogenous SerRS in HUVECs. The green signal corresponds to SerRS staining, whereas the blue corresponds to nuclear 4,6-diamidino-2-phenylindole (DAPI) staining. The picture was taken by confocal microscope in Z-mode. The cross-section at the yellow line is shown at the bottom. Representative SerRS nuclear localizations are marked with white arrowheads. (b) Cell fractionation assay confirming the nuclear localization of endogenous SerRS in both HUVEC and HEK 293 T cells. Nuclear (N) and cytoplasmic (C) extracts were analysed by western blot analysis. SerRS was detected by custom-made anti-SerRS antibody. Lamin A/C and α-tubulin were used as nuclear and cytoplasmic markers, respectively. (c) Confocal immunofluorescence microscopy showing that the NLS in UNE-S domain can facilitate the nuclear import of GFP protein in HEK 293 T and in HeLa cells. GFP protein is fused with the NLS sequence from human SerRS (GFP–NLS) at the C-terminus. The green signal corresponds to GFP or GFP–NLS, whereas the blue corresponds to nuclear DAPI staining. Scale bars in this figure correspond to 20 μm. Full size image Figure 2: Nuclear localization of SerRS. ( a ) Confocal immunofluorescence microscopy showing the nuclear localization of the endogenous SerRS in HUVECs. The green signal corresponds to SerRS staining, whereas the blue corresponds to nuclear 4,6-diamidino-2-phenylindole (DAPI) staining. The picture was taken by confocal microscope in Z-mode. The cross-section at the yellow line is shown at the bottom. Representative SerRS nuclear localizations are marked with white arrowheads. ( b ) Cell fractionation assay confirming the nuclear localization of endogenous SerRS in both HUVEC and HEK 293 T cells. Nuclear (N) and cytoplasmic (C) extracts were analysed by western blot analysis. SerRS was detected by custom-made anti-SerRS antibody. Lamin A/C and α-tubulin were used as nuclear and cytoplasmic markers, respectively. ( c ) Confocal immunofluorescence microscopy showing that the NLS in UNE-S domain can facilitate the nuclear import of GFP protein in HEK 293 T and in HeLa cells. GFP protein is fused with the NLS sequence from human SerRS (GFP–NLS) at the C-terminus. The green signal corresponds to GFP or GFP–NLS, whereas the blue corresponds to nuclear DAPI staining. Scale bars in this figure correspond to 20 μm. Full size image The potential NLS in UNE-S has the profile of a bipartite localization signal with two stretches of positively charged lysines that could be recognized by a nuclear transport protein [10] , [11] . To test its authenticity as an NLS, we added the corresponding sequence from human SerRS ( 482 KKQKK QHEGS KKK 494 ) to the carboxyl-terminus of the green fluorescent protein (GFP). The GFP–NLS fusion protein, when expressed in HeLa or HEK 293 T cells, predominantly localized to the nucleus ( Fig. 2c ). In contrast, the native GFP protein localized both to the nucleus and to the cytosol. These results show that the predicted NLS sequence in UNE-S is sufficient to direct nuclear localization. To establish whether the 482 KKQKK QHEGS KKK 494 NLS sequence is necessary for nuclear localization of SerRS, we deleted or mutated the NLS and compared the nuclear localization of the mutants with that of wild-type (WT) SerRS. As expected, the transfected WT protein was distributed in the nucleus of HEK 293 T cells ( Fig. 3a ). We then created two deletion mutations that removed either the entire UNE-S (Δ470-514) or only the region from the NLS to the C-terminus (Δ482-514). In contrast to the WT SerRS, both deletion constructs only appeared in the cytoplasm and had no detectable nuclear distribution ( Fig. 3a ). We also created mutants that replace lysine residues in the NLS with alanines. As the number of lysine substitutions increased, the amount of SerRS nuclear localization decreased. A single lysine mutant K493A had a slightly reduced nuclear localization (data not shown), but only trace amounts of the triple mutant K482A/K485A/K493A (designated as NLS mut ) were detected in the nucleus ( Fig. 3a ). These results strongly suggest that the predicted bipartite NLS in UNE-S is critical for the nuclear localization of SerRS. 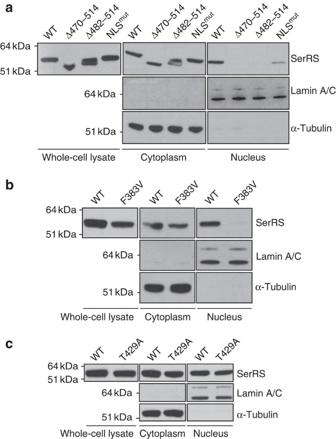Figure 3: UNE-S-dependent SerRS nuclear localization and its disruption by a mutation linked to vasculature abnormality. (a) Cell fractionation and mutagenesis studies showing that the predicted NLS within the UNE-S domain is responsible for the nuclear localization of SerRS. Subcellular localizations of the exogenously expressed SerRS proteins were detected by anti-flag tag polyclonal antibody. Deletion of the whole UNE-S domain (Δ470-514) or deletion from the NLS (Δ482-514) abolished the nuclear localization of SerRS. Triple point mutation within the NLS (K482A/K485A/K493A, designated as NLSmut) significantly reduced the nuclear localization. (b) Cell fractionation analysis demonstrating that the F383V mutant linked to vasculature abnormality in zebrafish is defective in nuclear localization. (c) Cell fractionation analysis confirms the intact nuclear localization of T429A SerRS. Figure 3: UNE-S-dependent SerRS nuclear localization and its disruption by a mutation linked to vasculature abnormality. ( a ) Cell fractionation and mutagenesis studies showing that the predicted NLS within the UNE-S domain is responsible for the nuclear localization of SerRS. Subcellular localizations of the exogenously expressed SerRS proteins were detected by anti-flag tag polyclonal antibody. Deletion of the whole UNE-S domain (Δ470-514) or deletion from the NLS (Δ482-514) abolished the nuclear localization of SerRS. Triple point mutation within the NLS (K482A/K485A/K493A, designated as NLS mut ) significantly reduced the nuclear localization. ( b ) Cell fractionation analysis demonstrating that the F383V mutant linked to vasculature abnormality in zebrafish is defective in nuclear localization. ( c ) Cell fractionation analysis confirms the intact nuclear localization of T429A SerRS. Full size image SerRS mutants are defective in nuclear localization Among the three different mutations in the SerRS gene ( SARS ) that are linked to zebrafish vasculature abnormalities, two were nonsense mutations resulting in a premature stop codon after Y401 or V420 [8] , [9] yielding C-terminal truncated SerRS proteins lacking UNE-S ( Fig. 1 ). Based on our data above, neither of these truncated proteins would be localized to the nucleus. The question remains on the third mutation, which results in a F383V substitution that is located ∼ 100 amino acids upstream of the NLS. Interestingly, this F383V substitution completely abolishes nuclear localization of SerRS ( Fig. 3b ). Thus, all three SerRS mutations linked to vasculature abnormalities in zebrafish would result in defective nuclear localization of SerRS. In contrast, the aminoacylation-defective T429A SerRS, which rescued the abnormal vascular phenotype, localizes to the nucleus as efficient as WT SerRS ( Fig. 3c ). The correlation between vasculature abnormality and the lack of SerRS nuclear localization strongly suggests that the role of SerRS in vascular development is dependent on the NLS embedded in UNE-S. Crystal structure analysis of human SerRS To understand how F383V affects nuclear localization, we determined the crystal structure of human SerRS at 2.9 Å resolution ( Fig. 4a and Supplementary Table S1 ). The human protein shares overall 81% sequence identity with the fish ortholog, and F383 is a strictly conserved residue from fish to humans ( Fig. 1 and Supplementary Fig. S1 ). Three independent homodimers of SerRS were found in the asymmetric unit of the crystal. While the conformation of the aminoacylation domain is almost the same for all three dimers in the asymmetric unit, the N-terminal tRNA-binding domains have more flexible structures ( Fig. 4b ). Interestingly, the C-terminal UNE-S domain (including the NLS) was mostly disordered in all six subunits, suggesting a dynamic conformation of the NLS that would enhance its accessibility to the nuclear transport machinery. F383 is located near the end of a β-strand (β10) that is part of the core seven-stranded antiparallel β-sheet (β1–β9–β10–β11–β13–β8–β7) of the aminoacylation domain, and spatially close to the active site and the flexible NLS ( Fig. 4a,c ). The side chain of F383 forms hydrophobic interactions with H170 and F316 to stabilize the β10–β11 hairpin as part of the central core ( Fig. 4c ). 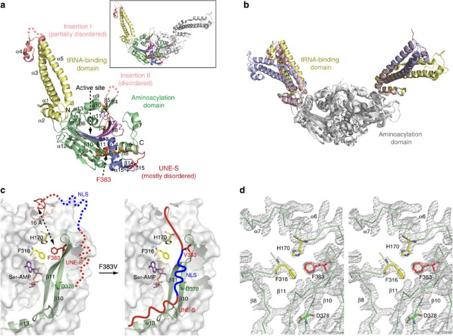Figure 4: Crystal structure of human SerRS and the hypothetic conformational change caused by F383V mutation. (a) Crystal structure of human SerRS showing one subunit of the dimer. Secondary structures are labelled on the ribbon diagram. Motifs 1, 2 and 3 within the aminoacylation domain are shown in orange, magenta and blue, respectively. Inset: SerRS dimer with the second subunit shown in grey. Dimerization is mediated through the aminoacylation domain. (b) Superposition of the three dimers of SerRS contained in each asymmetric unit. The aminoacylation domains are superimposed to show the flexibility of the N-terminal tRNA-binding domains. (c) Spatial location of residue F383. F383 is located in the loop region of the β10–β11 hairpin within the aminoacylation domain, and forms a hydrophobic pocket with residues H170 and F316. The hydrophobic pocket is close to the active site, which is indicated by a modelled Ser-AMP (aminoacylation reaction intermediate) molecule. The N-terminus of the UNE-S domain is located close to F383, and the rest of UNE-S including the NLS is disordered in the crystal structure. The F383V mutation might affect the conformation of UNE-S and obscure the NLS, as illustrated in a model of the F383V mutant shown on the right. (d) Stereo image of partial electron density around F383, F316, H170 and D378 (shown in sticks). The 2Fo-Fc electron density map at 1.5 σ is shown in grey, and the backbone traces of the structure are shown in light green. A stereo image of the electron density map surrounding F383 is shown in Figure 4d . We speculated that the F383V substitution would destabilize the hydrophobic core and, in some way, create an internal binding site for the NLS. As a result, the NLS would become less accessible, as illustrated in Figure 4c , and less able to facilitate nuclear localization. Figure 4: Crystal structure of human SerRS and the hypothetic conformational change caused by F383V mutation. ( a ) Crystal structure of human SerRS showing one subunit of the dimer. Secondary structures are labelled on the ribbon diagram. Motifs 1, 2 and 3 within the aminoacylation domain are shown in orange, magenta and blue, respectively. Inset: SerRS dimer with the second subunit shown in grey. Dimerization is mediated through the aminoacylation domain. ( b ) Superposition of the three dimers of SerRS contained in each asymmetric unit. The aminoacylation domains are superimposed to show the flexibility of the N-terminal tRNA-binding domains. ( c ) Spatial location of residue F383. F383 is located in the loop region of the β10–β11 hairpin within the aminoacylation domain, and forms a hydrophobic pocket with residues H170 and F316. The hydrophobic pocket is close to the active site, which is indicated by a modelled Ser-AMP (aminoacylation reaction intermediate) molecule. The N-terminus of the UNE-S domain is located close to F383, and the rest of UNE-S including the NLS is disordered in the crystal structure. The F383V mutation might affect the conformation of UNE-S and obscure the NLS, as illustrated in a model of the F383V mutant shown on the right. ( d ) Stereo image of partial electron density around F383, F316, H170 and D378 (shown in sticks). The 2Fo-Fc electron density map at 1.5 σ is shown in grey, and the backbone traces of the structure are shown in light green. Full size image Solution structure shows the effect of F383V on UNE-S To compare the conformational dynamics of the NLS between the WT and F383V SerRS in solution, we carried out hydrogen–deuterium exchange analysis monitored by mass spectrometry (HDX-MS). The rate and level of hydrogen–deuterium exchange of each digested peptide throughout the protein are directly related to its local conformation: more solvent-accessible and less H-bonded peptides exhibit faster and greater deuterium exchange than less solvent-accessible and more H-bonded ones [12] . The SerRS proteins in this work exhibited the EX2 exchange regime, which is typical for most proteins in physiological conditions. By comparing the level of hydrogen–deuterium exchange of the same peptide segments in the WT and F383V SerRS, a difference map was constructed ( Supplementary Fig. S2 ). The peptide covering the F383V mutation site (E380-L392) is the only area on the protein that exhibits a dramatic increase in HDX (41% over WT SerRS) ( Supplementary Fig. S2 and Fig. 5a ), presumably because of the weakened hydrophobic core caused by the mutation. Remarkably, also as a result of the F383V mutation, the NLS region shows the most dramatic decrease in HDX (64% below WT SerRS), indicating that it is stabilized in the mutant. This result is consistent with our hypothesis that the NLS becomes less accessible in the F383V mutant ( Figs 4c and 5a ). 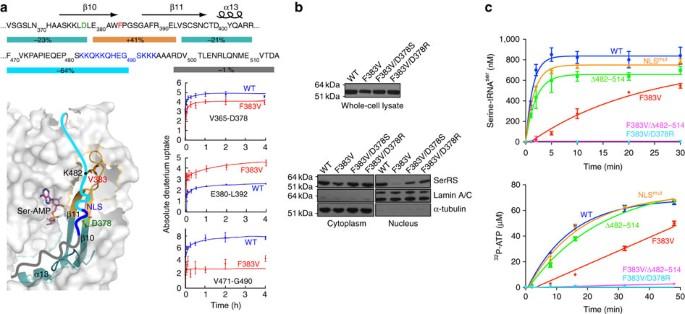Figure 5: Structural and functional analysis of WT and F383V SerRS. (a) HDX-MS analysis of WT and F383V human SerRS proteins in solution showing that the NLS is conformationally buried in F383V SerRS. The regions associated with major deuterium uptake differences between WT and F383V SerRS are mapped on the primary sequence and on the crystal structure of human SerRS with the same colour coding. The percentage difference of deuterium incorporation indicated under the primary sequence is calculated from the hydrogen–deuterium exchange after 1 h for F383V mutant relative to WT SerRS. Deuterium uptake time-course curves for representative peptides are shown on the right. (b) Cell fractionation experiment showing that substitution of D378 with S or R rescues the nuclear localization deficiency of F383V SerRS. (c) Aminoacylation and ATP-PPi exchange assays showing that the NLS is dispensable for aminoacylation and the F383V mutant remains partially active. The partial activity of F383V SerRS is completely lost when the NLS is deleted or released by the second mutation D378R. Error bars represent the s.e.m of triplicate experiments. Figure 5: Structural and functional analysis of WT and F383V SerRS. ( a ) HDX-MS analysis of WT and F383V human SerRS proteins in solution showing that the NLS is conformationally buried in F383V SerRS. The regions associated with major deuterium uptake differences between WT and F383V SerRS are mapped on the primary sequence and on the crystal structure of human SerRS with the same colour coding. The percentage difference of deuterium incorporation indicated under the primary sequence is calculated from the hydrogen–deuterium exchange after 1 h for F383V mutant relative to WT SerRS. Deuterium uptake time-course curves for representative peptides are shown on the right. ( b ) Cell fractionation experiment showing that substitution of D378 with S or R rescues the nuclear localization deficiency of F383V SerRS. ( c ) Aminoacylation and ATP-PPi exchange assays showing that the NLS is dispensable for aminoacylation and the F383V mutant remains partially active. The partial activity of F383V SerRS is completely lost when the NLS is deleted or released by the second mutation D378R. Error bars represent the s.e.m of triplicate experiments. Full size image Structure-based design of second-site revertant of F383V We next wanted to determine the F383V-induced internal binding site for the NLS. By analysing the surface electrostatic potential of SerRS, three negatively charged sites were identified as potential binding sites for the positively charged NLS. Those sites are spatially adjacent to both the F383V mutation site and the partially resolved UNE-S in the crystal structure. As shown in Supplementary Figure S3a,b , site I contains four negatively charged residues (D148, E149, E150 and D152), site II contains D178, E181 and E183, while site III contains D378, E380 and E391. Among them, site III is the closest to the F383V mutation site ( Supplementary Fig. S3b ). If some of those negatively charged residues are important for NLS binding, their substitution with neutral or positively charged residues would release the NLS and restore nuclear localization. To identify the NLS-binding site on F383V SerRS, we created mutations within each site (I or II or III) on top of the F383V background. While mutations within sites I and II did not have any effect on nuclear localization ( Supplementary Fig. S3c ), a double mutation within site III (D378S/E380G) partially rescued the nuclear localization defect of F383V ( Supplementary Fig. S3c ). The rescue effect was mostly contributed by the D378S mutation alone, while substitution of D378 with a positively charged arginine provided further rescue ( Fig. 5b ). These results suggest that D378 has a major role in tethering the NLS in F383V SerRS, and that this tethering effect is largely dependent on electrostatic interactions. Consistently, as a result of the NLS binding, the D378-containing peptide (V365-D378) exhibited a 23% decrease in HDX in F383V SerRS relative to the WT protein ( Fig. 5a ). Possibly, as the F383V mutation increases the conformational dynamics of the loop region of the β10–β11 hairpin ( Fig. 5a ), a binding groove is opened up near the hydrophobic core to accommodate the NLS that is then tethered by D378. UNE-S is dispensable for SerRS aminoacylation Previous studies showed that the vasculature defect in zebrafish was rescued by the expression of an enzymatically inactive SerRS. This result suggested that the role of SerRS in vascular development is separate from its role in protein synthesis. Therefore, the NLS, if related to vascular development, might not be involved in the enzymatic activity of SerRS. To investigate this point, we studied the two-step aminoacylation reaction. In the first step, serine is condensed with ATP to from seryl-adenylate (Ser-AMP). In the second step, serine is transferred from Ser-AMP to tRNA Ser . Using standard assays, we showed that, indeed, mutation or deletion of the UNE-S did not affect either of the two steps of the aminoacylation reaction ( Fig. 5c and Supplementary Table S2 ). However, the F383V mutation reduced the catalytic activity of SerRS ( Fig. 5c ). This might be due to the proximity of F383 to the active site, and the disturbance to the hydrophobic core next to the active site caused by the F to V substitution, as seen in the HDX experiment ( Fig. 5a ). Remarkably, deletion of the NLS, which had no effect on the aminoacylation activity of WT SerRS, completely abolished the residual enzymatic activity of F383V SerRS ( Fig. 5c ). The second-site mutation D378R, which reverts the nuclear localization defect of F383V, also completely abolished the enzymatic activity of F383V SerRS. These observations further support a strong interplay between the NLS and D378 in the F383V mutant. Presumably, through the interaction with D378, the NLS helps to partially restore the destabilized active site resulting from the F383V mutation. Removal of this interaction, either by deletion of the NLS or by mutation of D378, abrogates the restoration effect. Role of UNE-S in vascular development in the zebrafish To confirm a functional link between the NLS and vascular development in a vertebrate model, we tested the rescue of vascular abnormality in zebrafish by various SerRS mutants. A fish model for vasculature abnormalities was created by injecting an antisense morpholino (MO) directed against SerRS [8] . Consistent with the previous report by Fukui et al . [8] , we show that injection of SerRS-MO results in abnormal intersegmental vessel (ISV) branching in 50.8% ( n =96 out of 189) of morphants, in contrast to 1.4% ( n =3 out of 207) in uninjected controls ( Fig. 6a and Table 1 ). Co-injection of human SerRS mRNA efficiently rescued the abnormal ISV branching (8.4%; n =16 out of 190) in SerRS morphants ( Fig. 6a and Table 1 ). 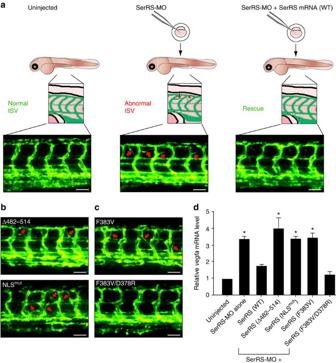Figure 6: Rescue experiments in zebrafish demonstrating the role of UNE-S in vascular development. (a) Illustration of the phenotype rescue experiment in zebrafish. The SerRS morpholino (SerRS-MO,∼5 ng per embryo) was injected into the yolk of zebrafish embryos (1- to 2-cell stage) to produce a model of intersegmental vessel (ISV) abnormality. Co-injection of SerRS-MO with the WT human SerRS mRNA (∼250 pg per embryo) rescued the aberrant ISV branching. The ISV development is recorded at 72 h post fertilization and the abnormal ISV branches are indicated by red arrows. (b) Co-injection of SerRS-MO with the NLS-deleted Δ482-514 or NLSmuthuman SerRS mRNA did not rescue the aberrant ISV branching. (c) Co-injection of SerRS-MO with F383V human SerRS mRNA did not, whereas with F383V/D378R SerRS mRNA did, rescue the aberrant ISV branching. (d) The effect of SerRS nuclear localization on VEGFA transcription. Semiquantitative RT–PCR analysis to evaluatevefgamRNA levels in 72-hpf zebrafish embryos injected with SerRS-MO alone or SerRS-MO together with WT or mutant human SerRS mRNAs. RelativevegfamRNA levels represented as fold increase (mean±s.e.m.,n=3, *P<0.05 (Student'st-test)) over uninjected control samples, after normalization to the levels ofβ-actinmRNA. Scale bars in this figure correspond to 100 μm. Figure 6: Rescue experiments in zebrafish demonstrating the role of UNE-S in vascular development. ( a ) Illustration of the phenotype rescue experiment in zebrafish. The SerRS morpholino (SerRS-MO, ∼ 5 ng per embryo) was injected into the yolk of zebrafish embryos (1- to 2-cell stage) to produce a model of intersegmental vessel (ISV) abnormality. Co-injection of SerRS-MO with the WT human SerRS mRNA ( ∼ 250 pg per embryo) rescued the aberrant ISV branching. The ISV development is recorded at 72 h post fertilization and the abnormal ISV branches are indicated by red arrows. ( b ) Co-injection of SerRS-MO with the NLS-deleted Δ482-514 or NLS mut human SerRS mRNA did not rescue the aberrant ISV branching. ( c ) Co-injection of SerRS-MO with F383V human SerRS mRNA did not, whereas with F383V/D378R SerRS mRNA did, rescue the aberrant ISV branching. ( d ) The effect of SerRS nuclear localization on VEGFA transcription. Semiquantitative RT–PCR analysis to evaluate vefga mRNA levels in 72-hpf zebrafish embryos injected with SerRS-MO alone or SerRS-MO together with WT or mutant human SerRS mRNAs. Relative vegfa mRNA levels represented as fold increase (mean±s.e.m., n =3, * P <0.05 (Student's t -test)) over uninjected control samples, after normalization to the levels of β-actin mRNA. Scale bars in this figure correspond to 100 μm. Full size image Table 1 Statistics of ISV abnormal branching rescued by WT or mutant human SerRS mRNA injection. Full size table In contrast, Δ482-514, NLS mut and F383V SerRS, which we showed to be defective in nuclear localization ( Fig. 3a,b ), could not rescue the aberrant ISV branching ( Fig. 6b,c and Table 1 ). Abnormal ISV branching was observed in 44.6% ( n =79 out of 177), 51.0% ( n =77 out of 151) and 45.1% ( n =69 out of 153) of SerRS morphants injected with Δ482-514, NLS mut and F383V SerRS mRNA, respectively. These results strongly suggested that the NLS introduced by UNE-S is essential for vascular development. To further establish this conclusion, the rationally designed second-site revertant that restores nuclear localization by a compensatory substitution distal to the NLS was tested. Strikingly, the double mutant F383V/D378R SerRS mRNA rescued the abnormal ISV branching defects (8.5%; n =13 out of 153) with efficiency comparable to that of the WT mRNA ( Fig. 6c and Table 1 ). The result further demonstrated the critical link of the NLS and UNE-S with vasculature development. The critical role of the NLS in the UNE-S domain indicates a specific function for SerRS in the nucleus of vertebrate cells. Fukui et al . [8] reported that the ko095 SerRS mutant zebrafish had increased expression of vegfa , which was suppressed by microinjection of the aminoacylation-defective T429A SerRS mRNA, suggesting that the noncanonical role of SerRS is related to negative regulation of vegfa expression [8] . Consistently, Herzog et al . [9] showed that inhibition of VEGF signalling rescued aberrant dilatation of the aortic arch vessels in SerRS mutant zebrafish. To address the question of whether the function of SerRS in regulating VEGFA was also linked to UNE-S, we examined vegfa mRNA levels in fish embryos obtained from our previous experiments. The observed vascular abnormality was clearly coincident with upregulation of vegfa expression. Compared with the uninjected group, embryos injected with the SerRS MO have more than a threefold increase in vegfa mRNA level ( Fig. 6d ). This increase was largely suppressed when WT or F383V/D378R SerRS mRNA was co-injected with the SerRS MO ( Fig. 6d ). In contrast, co-injection of nuclear localization-defective Δ482-514 or NLS mut or F383V SerRS did not suppress vegfa expression. Thus, regulation of vegfa expression was also dependent on UNE-S and the nuclear localization of SerRS. This observation suggested that the function of SerRS in the nucleus is related to VEGFA regulation. Blood vessel formation, or vasculogenesis, is one of the hallmarks of vertebrate development. During the invertebrate-to-vertebrate transition, the open circulatory systems, where blood is pumped by the heart into the body cavities, of invertebrates evolved into the advanced closed circulatory systems, where vessels are developed to carry the blood to nourish organs and tissues. As the invertebrate-to-vertebrate transition coincides with the appearance of UNE-S, and because UNE-S is shown here to be essential for vascular development, acquisition of UNE-S may have a role in the establishment of the closed circulatory systems of vertebrates. It is worth noting that, as the tree of life ascended from bacteria to lower and higher eukaryotes, new domains or motifs were added to aaRSs in a progressive and accretive manner [6] . In the case of SerRSs, the acquisition consists of extensions beyond the C-termini of the bacterial orthologs ( Fig. 1 and Supplementary Fig. S1 ). SerRSs from basal eukaryotes have short C-terminal extensions that, as shown for Saccharomyces cerevisiae , while appearing to be important for stability of the synthetase in vitro and in vivo , are dispensable for aminoacylation [13] . However, in going through the transition from invertebrates to vertebrates, the C-terminus of SerRS was significantly expanded into the UNE-S domain. While it remains not important for aminoacylation ( Fig. 5c ), the expansion included the appearance of a robust NLS. Our work showed that, because of the NLS brought in by UNE-S, this novel appended domain can mobilize SerRS for translocation from the cytosol to the nucleus—a function that is orthogonal to aminoacylation. Once in the nucleus, SerRS has the additional function of regulating expression of VEGFA, a key regulator of vascular development, most likely at the level of transcription. This nuclear activity of SerRS is in some ways reminiscent of the reported activity of LysRS, which regulates transcription factors MITF and USF2 that alter expression of target genes in response to allergic stimulation [14] , [15] , [16] . From another aspect, the role of nuclear SerRS mirrors that of the bifunctional GluProRS, which in response to interferon-gamma stimulation, silences translation of VEGFA mRNA in the cytoplasm [17] . Thus, an increasing literature has reported the role of aaRSs in regulating gene expression. In this regard, the work reported here is the first to show how an appended domain mobilizes a synthetase for an ex-translational role related to gene transcription. A lysine-rich peptide derived from a putative NLS sequence at the N-terminus of Lupinus luteus GlnRS was shown to interact with DNA and was suggested to potentially regulate gene expression [18] . The NLS within the UNE-S domain of SerRS is also lysine-rich and has a flexible conformation, as revealed in our crystal structure of human SerRS (which is the first structure of a vertebrate SerRS). This flexibility was further demonstrated through the UNE-S conformational switch induced by the F383V mutation. As flexible protein motifs are known to adapt by induced fit to specific DNA sequence targets, UNE-S may not only mobilize SerRS for nuclear localization but also facilitate interactions with potential targets in the nucleus. Given that almost all aaRSs have their own distinct elaborations with new domains, our work provides further motivation to discover and understand the function and significance of other synthetase domain accretions in higher organisms. Among them, the N-terminal WHEP domain of TrpRS is of particular interest, because it also appears during the transition from invertebrates to vertebrates and has been shown to regulate the anti-angiogenic activity of human TrpRS [19] , [20] . Confocal immunofluorescence microscopy To detect SerRS subcellular localization, HUVEC cells were seeded on cover slips and grown overnight. After fixing and permeabilization, cells were stained with custom-made rabbit anti-SerRS antibody (1 μg ml −1 ) followed by Aflex Fluor 488 (green) goat anti-rabbit IgG (at 1:1000 dilution) and 4,6-diamidino-2-phenylindole (1 μg ml −1 ). The photos of the cells were taken with a Bio-Rad (Zeiss) Radiance 2100 Rainbow laser scanning confocal microscope in Z-mode (×60 oil objective). Nuclear fractionation analysis Human SerRS gene was cloned from HEK293 T cell by RT–PCR and then inserted into pFLAG-CMV2 vector (Sigma-Aldrich) with an N-terminal flag tag. Mutant SerRS constructs were generated by site-directed mutagenesis and transfected into HEK 293 T cells. Cells were harvested after 24 h, and the cytoplasmic and nuclear fractions were separated and extracted by using NE-PER Nuclear and Cytoplasmic Extraction Kit (Thermo Scientific). Exogenously expressed SerRS proteins were detected by western blot analysis using anti-flag polyclonal antibody (Sigma-Aldrich). Protein overexpression and crystallization Human SerRS gene was also cloned into pET20b vector (Novagen) with a C-terminal 6×His tag and overexpressed in E. coli BL21 (DE3) cells. SerRS protein was purified in tandem by Ni-NTA affinity (Qiagen) and HiLoad 26/10 Phenyl Sepharose High Performance columns (GE Healthcare). The purified protein was stored in 25 mM Tris-Cl pH 8.0, 0.1 M ammonium sulphate before setting up for high-throughput crystallization using Mosquito liquid transfer robot (TTP Labtech). By use of sitting-drop vapour diffusion method, crystals were obtained at room temperature by mixing 0.1 μl human SerRS (20 mg ml −1 , pre-incubated with 5 mM ATP and 10 mM MgCl 2 ) and 0.1 μl reservoir solution (20% PEG 3350, 0.2 M tri-sodium citrate pH 7.0) equilibrated against 70 μl reservoir solution. Crystal data collection and structure determination Crystals were cryoprotected with 15% glycerol added to the reservoir solution and flash frozen with liquid nitrogen. A 2.9 Å resolution data set was collected at 100 K on beamline BL7-1 at Stanford Synchrotron Radiation Laboratory with an ADSC Q315 detector. The crystal belongs to space group P2 1 2 1 2 1 with unit cell dimensions a =116.80 Å, b =189.42 Å and c =230.59 Å. Diffraction data were processed, integrated and scaled with HKL2000 [21] . The structure of human SerRS was solved by molecular replacement using Pyrococcus horikoshii SerRS (PDB 2ZR3) [22] structure as search model in program PHASER [23] from the CCP4 package [24] . Three homodimers of SerRS were found in one asymmetric unit with ∼ 55% solvent content [25] . Iterative model building and refinement were performed using Coot [26] and Phenix [27] with 83% of the polypeptide chains resolved in the final model with R work of 20.8% and R free of 25.7% at 2.9 Å resolution. HDX and mass spectrometry SerRS mutant proteins were overexpressed and purified as described for the WT protein, and stored in 25 mM HEPES pH 7.5 and 150 mM NaCl. To initiate the HDX reaction, 5 μl of SerRS protein (WT or F383V mutant) was incubated with 45 μl of DPBS buffer in D 2 O (2.6 μM final concentration) for 0.5, 1, 2, 4, 8, 15, 30, 60, 120 or 240 min, followed by simultaneous quench and proteolysis by addition of protease type XIII solution (threefold dilution from a saturated solution) in 1.0% formic acid, 40 mM TCEP and 4 M urea [28] . The digested peptide fragments were separated by a fast LC gradient through a ProZap C 18 column (Grace Davison, 1.5 μm, 500 Å, 2.1×10 mm) to minimize back exchange [29] . A post-column splitter reduced the LC eluent flow rate to ∼ 400–500 nl min −1 for efficient microelectrospray ionization (micro-ESI) [30] . Microelectrosprayed HDX samples were directed to a custom-built hybrid linear trap quadrupole 14.5-Tesla FT-ICR mass spectrometer (ThermoFisher, San Jose, CA) for accurate mass measurement [31] . The total data acquisition period for each sample was 6 min. All experiments were performed in triplicate. Data were analysed with a custom analysis package [32] and a Python program [33] . Time-course deuterium incorporation levels were generated by an MEM fitting method [34] . Active site titration assay Active site titration assay was performed in 100 mM HEPES pH 7.5, 20 mM KCl, 10 mM MgCl 2 , 50 μM ATP, 22.2 nM [γ- 32 P]-ATP, 20 mM L -serine, 2 μg ml –1 pyrophosphatase (Roche) and 2 mM dithiothreitol (DTT) as previously described [35] to determine the concentration of active enzymes. ATP-PPi exchange assay ATP-PPi exchange assay was performed with 0.5 μM SerRS (WT or mutants) in 100 mM HEPES pH 7.5, 20 mM KCl, 10 mM MgCl 2 , 2 mM ATP, 500 μM L -serine, 1 mM Na-PPi and 0.07 mCi Na- 32 PPi and 2 mM DTT as described [35] . The kinetics parameters of ATP and serine for each enzyme (WT at 65 nM; F383V at 135 nM; Δ482–514 at 73 nM; NLS mut at 91 nM) were determined by varying the ATP and serine concentrations, respectively, while saturating the concentration of the other substrate. In vitro transcription and purification of tRNA ser The tRNA ser (AGA) coding sequence was cloned into pUC18 vector with a T7 promoter sequence at the 5′-end and a BstNI restriction enzyme site at the 3′-end to allow generation of a linear template that would give the correct 3′-CCA end in the tRNA transcript. In vitro transcription was performed in 40 mM Tris-Cl pH 8.0, 25 mM NaCl, 20 mM MgCl 2 , 1 mM spermidine, 2 μg ml −1 pyrophosphatase, 0.1 mg ml −1 bovine serum albumin, 5 mM DTT, NTPs with T7 polymerase and BstNI-linearized DNA template at 37°C. The tRNA transcript was purified by Mono Q HR5/5 anion exchange column (GE Healthcare). The purified tRNA was annealed by heating up to 95°C and then slowly cooled to room temperature. Aminoacylation assay Aminoacylation assays were performed as described [35] with 50-nM enzyme in 50 mM HEPES pH 7.5, 20 mM KCl, 10 mM MgCl 2 , 4 mM ATP, 2 μM [ 3 H]- L -serine, 20 μM L -serine, 2 mM DTT, 0.1 mg ml −1 bovine serum albumin, 4 μg ml −1 pyrophosphatase (Roche) and 1 μM tRNA ser transcript. Kinetics parameters of tRNA ser were determined by varying the tRNA concentration from 0.1× ∼ 10× K m for each enzyme. In vivo studies in zebrafish Transgenic Tg ( Fli1a: EGFP ) fish were maintained at 28.5°C under continuous water flow and filtration with automatic control for a 14:10 h light/dark cycle. The night before injection, male and female fish were placed in a 1-l tank containing fish mating cage with an inner mesh and divider. Zebrafish embryos were obtained from natural spawning by removing the divider and stimulating with light. The embryos were kept at 28.5°C before and after microinjection. The SerRS MO was injected into the yolk of 1- to 2-cell stage embryos at the dosage of 4 ∼ 5 ng per embryo. The SerRS morpholino (5′-AG GAGAATGTGAACAAACCTGACAC-3′) was purchased from Gene Tools, LLC (Philomath, OR, USA). Capped mRNAs of WT or various human SerRS mutants were synthesized by use of the mMESSAGE mMACHINE (Ambion). Synthetic mRNAs were injected into the 1-cell stage embryos together with SerRS-MO at a dosage of ∼ 250 pg per embryo. After injection, embryos were incubated in E3 embryo medium supplemented with 0.003% 1-phenyl-2-thiourea at 28.5°C to prevent pigment formation. Embryos were anesthetized with 0.168 mg ml −1 tricaine (Sigma-Aldrich), mounted in 2% methylcellulose and photographed with a Nikon fluorescent microscope (AZ100) equipped with a Nikon CCD camera (Qimaging Retiga 2000R). All the experiments involving zebrafish had been conducted according to the guidelines established by the Institutional Animal Care and Use Committee (IACUC) at The Scripps Research Institute, IACUC approval number 09-0009. Reverse transcription PCR Seventy-two hours after injection, ten zebrafish embryos from each group were collected for total RNA extraction using Trizol reagent (Invitrogen) according to the manufacturer's instruction. The total RNAs (1 μg for each group) were reverse transcribed by using M-MLV reverse transcriptase (Promega) and oligo dT(20) as the primer. The reverse transcription products were then used as templates for PCR reaction using the Taq DNA polymerase (Fermentas). The sequences of the primers for zebrafish vegfa are: 5′-GGCTCTCCTCCATCTGTCTGC-3′ (forward) and 5′-CAGTGGTTTTCTTTCTTTGCTTTG-3′ (reverse). The sequences of the primers for zebrafish β-actin are: 5′-TCACCACCACAGCCGAAAGAG-3′ (forward) and 5′-GTCAGCAATGCCAGGGTACAT-3′ (reverse). Each PCR cycle includes denaturation at 95°C for 30 s, annealing at 60°C for 20 s and elongation at 72°C for 20 s. We performed 28 cycles of PCR for the vegfa gene and 18 cycles for the β-actin gene. The PCR products were then analysed by agarose gel electrophoresis and visualized by ethidium bromide staining. The density of each band was semiquantificated on the gel image using Multi Gauge V3.0 software (Fujifilm). The relative expression levels of vegfa were determined after normalization to β-actin. Accession codes: The atomic coordinates for the SerRS crystal structure have been deposited in the Protein Data Bank under accession code 3VBB . How to cite this article: Xu, X. et al . Unique domain appended to vertebrate tRNA synthetase is essential for vascular development. Nat. Commun. 3:681 doi: 10.1038/ncomms1686 (2012).